Effect of iron oxidation state on the electrical conductivity of the Earth’s lower mantle Iron can adopt different spin states in the lower mantle. Previous studies indicate that the dominant lower-mantle phase, magnesium silicate perovskite (which contains at least half of its iron as Fe 3+ ), undergoes a Fe 3+ high-spin to low-spin transition that has been suggested to cause seismic velocity anomalies and a drop in laboratory-measured electrical conductivity. Here we apply a new synchrotron-based method of Mössbauer spectroscopy and show that Fe 3+ remains in the high-spin state in lower-mantle perovskite at conditions throughout the lower mantle. Electrical conductivity measurements show no conductivity drop in samples with high Fe 3+ , suggesting that the conductivity drop observed previously on samples with high Fe 2+ is due to a transition of Fe 2+ to the intermediate-spin state. Correlation of transport and elastic properties of lower-mantle perovskite with electromagnetic and seismic data may provide a new probe of heterogeneity in the lower mantle. Pressure-induced spin transitions (that is, changes in the pairing of electrons in the atomic orbitals) of iron in lower-mantle minerals can significantly influence mantle properties and dynamics. One factor that strongly influences the potential for a particular iron species to undergo a spin transition is its surrounding crystallographic environment. The structure of the Earth’s most abundant phase, iron-containing magnesium aluminium silicate perovskite (hereafter referred to as FeAlPv), contains two sites, a large 8–12 coordinated site (‘A’) and a smaller octahedral site (‘B’). At least half of the iron in FeAlPv in the lower mantle is expected to be Fe 3+ (refs 1 , 2 , 3 ), which can occupy either the A site or the B site. The A site is additionally occupied primarily by Mg 2+ and Fe 2+ , and the B site by Si 4+ and Al 3+ . Previous studies of spin transitions of Fe 3+ in FeAlPv are broadly consistent, and have shown that a high-spin (HS) (five unpaired d electrons) to low-spin (LS) (one unpaired d electron) transition is predicted when Fe 3+ occupies the B site, whereas Fe 3+ A (that is, Fe 3+ in the A site) is predicted to remain in the HS state at all pressures throughout the lower mantle [4] , [5] , [6] , [7] , [8] , [9] , and several studies have additionally predicted exchange of Fe 3+ from the A to the B site at pressures above the HS–LS transition [6] , [8] , [9] . The drop in electrical conductivity observed with increasing pressure [10] , [11] , [12] has generally been attributed to a HS–LS transition of Fe 3+ . However, there are also reports of a transition of Fe 2+ in FeAlPv that starts above ~30 GPa, although there is disagreement as to whether it involves a HS (four unpaired d electrons) to intermediate-spin (IS) (two unpaired d electrons) transition [13] , [14] , [15] or simply a structural modification of the local atomic environment [16] . Detecting spin transitions in FeAlPv presents a significant challenge. X-ray emission spectroscopy provides information on the bulk spin number, but cannot separate individual contributions. In contrast, energy-domain 57 Fe Mössbauer spectroscopy generally enables an unambiguous resolution of all hyperfine parameters, which can be used to infer spin states; however, high-pressure measurements using conventional radioactive point sources require extremely long counting times (generally more than 1 week per spectrum). Third-generation synchrotron sources offer a solution in the form of time-domain Mössbauer spectroscopy (that is, nuclear forward scattering); however, this method is not well suited to materials with a large number of components (such as FeAlPv) because of the resulting complex spectra. To solve this problem, we have developed an energy-domain synchrotron Mössbauer source (SMS) that offers a number of advantages over conventional Mössbauer spectroscopy: high brilliance and a nearly fully resonant emitted beam that can be focused to a spot of only a few microns diameter, and in contrast to time-domain spectroscopy, spectra that deliver direct and unambiguous information [17] , [18] . Therefore, SMS spectroscopy allows for rapid measurement of energy-domain Mössbauer spectra under extreme conditions with a quality generally sufficient to unambiguously deconvolute even highly complex spectra. In this study, involving SMS measurements over a wide range of FeAlPv compositions with varying Fe 3+ /ΣFe, we show that Fe 3+ remains in the HS state at pressure–temperature conditions relevant for the lower mantle, whereas Fe 2+ undergoes the same transition observed in previous experiments [13] , [14] , [15] . Combined with new high-pressure high-temperature electrical conductivity data on Fe 3+ -rich FeAlPv, we suggest that the drop in conductivity observed in previous experiments [10] , [11] , [12] is due to the hotly disputed HS to IS transition in Fe 2+ . These results may place improved constraints on the interpretation of lower-mantle electrical conductivity profiles as well as of joint inversions of electromagnetic and seismic data, potentially providing a new probe for heterogeneity in the lower mantle. Sample synthesis and characterization We studied four different FeAlPv samples: Mg 0.6 Fe 0.4 Si 0.63 Al 0.37 O 3 sample no. 1 (~80% Fe 3+ /ΣFe); Mg 0.6 Fe 0.4 Si 0.63 Al 0.37 O 3 sample no. 2 (~70% Fe 3+ /ΣFe); Mg 0.83 Fe 0.2 Al 0.06 Si 0.91 O 3 (~50% Fe 3+ /ΣFe) (sample no. 3); and Mg 0.94 Fe 0.06 SiO 3 (~20% Fe 3+ /ΣFe) (sample no. 4). 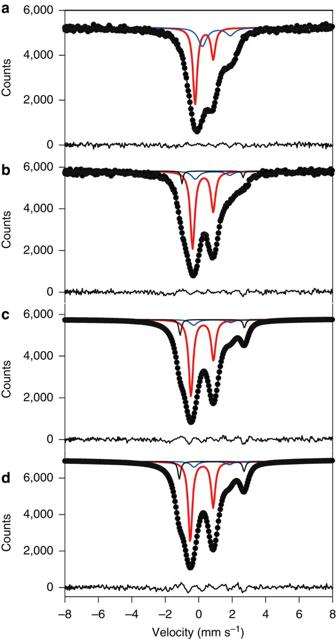Figure 1: Influence of pressure on SMS spectra of FeAlPv. Room temperature spectra are shown for Mg0.6Fe0.4Si0.63Al0.37O3perovskite sample no. 1 at the following pressures: (a) 2.5 GPa; (b) 37.9 GPa; (c) 67 GPa; and (d) 93 GPa. The data were fit to one Fe3+doublet (red) and two Fe2+doublets (blue and black), and the fit residual is shown below each spectrum. Area asymmetry is due to preferred orientation of the sample, and the velocity scale is given relative to α-iron. Details of sample synthesis and characterization are summarized in Table 1 . Table 1 Experimental details and FeAlPv compositions. Full size table Single-crystal X-ray refinements and crystal chemical calculations show that Fe 3+ occupies predominantly the A site of the perovskite structure in all of our samples. Full structural refinements of a single crystal of FeAlPv synthesized using identical starting materials and experimental procedure to (Mg 0.6 Fe 0.4 )(Si 0.63 Al 0.37 )O 3 perovskite (sample no. 1 and 2) (with the exception that iron was not 57 Fe enriched) using in situ X-ray diffraction data collected in a diamond anvil cell (DAC) at pressures up to 80 GPa and temperatures over 1700 K (ref. 19 ) showed that both Fe 2+ and Fe 3+ occupy the A site exclusively at all conditions studied. We therefore expect a similar site distribution for sample no. 1 and 2 in the current study. For Mg 0.83 Fe 0.2 Al 0.06 Si 0.91 O 3 perovskite (sample no. 3), electron microprobe data combined with results from Mössbauer spectroscopy gave the following site distribution: [Mg 0.828(18) Fe 2+ 0.104(13) Fe 3+ 0.075(13) ] A [Si 0.911(23) Al 0.059(2) Fe 3+ 0.029(13) ] B O 3 . Iron occupies predominantly the A site, although the presence of a small amount of Fe 3+ on the B site cannot be ruled out within the uncertainty of the data. For (Mg 0.94 Fe 0.06 )SiO 3 perovskite (sample no. 4), we selected a single crystal from the same high-pressure synthesis run and conducted a full structural refinement using SHELXL97 software on X-ray diffraction data collected at ambient conditions using an Oxford Diffraction Xcalibur diffractometer. Details of the structural refinement will be published elsewhere. The refinement showed that all iron occupied the A site exclusively. Electron microprobe data combined with results from Mössbauer spectroscopy gave the following site distribution: [Mg 0.946(17) Fe 2+ 0.045(12) Fe 3+ 0.008(3) ] A [Si 0.997(16) Fe 3+ 0.003(3) ] B O 3 , which means that a small amount of Fe 3+ on the B site cannot be ruled out within the uncertainty of the electron microprobe and Mössbauer data. SMS spectroscopy We collected SMS spectra at room temperature and pressures up to 122 GPa using DACs, with or without laser annealing of the samples. SMS spectra of Mg 0.6 Fe 0.4 Si 0.63 Al 0.37 O 3 perovskite (sample no. 1), which contains iron dominantly as Fe 3+ , are extremely well resolved ( Fig. 1 ). We fit the data to three quadrupole doublets, one assigned to Fe 3+ and two assigned to Fe 2+ based on their centre shifts. Visually there appears to be no change to the Fe 3+ doublet over the entire pressure range ( Fig. 1 and Supplementary Fig. S1 ). Figure 1: Influence of pressure on SMS spectra of FeAlPv. Room temperature spectra are shown for Mg 0.6 Fe 0.4 Si 0.63 Al 0.37 O 3 perovskite sample no. 1 at the following pressures: ( a ) 2.5 GPa; ( b ) 37.9 GPa; ( c ) 67 GPa; and ( d ) 93 GPa. The data were fit to one Fe 3+ doublet (red) and two Fe 2+ doublets (blue and black), and the fit residual is shown below each spectrum. Area asymmetry is due to preferred orientation of the sample, and the velocity scale is given relative to α-iron. Full size image The hyperfine parameters (centre shift and quadrupole splitting (QS)) for Fe 3+ in all samples are the same within experimental error, and there is no change in Fe 3+ /ΣFe for individual samples over the entire pressure range of the experiment ( Fig. 2 ). The hyperfine parameters of the Fe 3+ doublet are consistent with the HS state [20] , and their smooth variation with pressure indicates that Fe 3+ does not undergo any spin transitions within the entire pressure range. Notably, the QS value proposed for LS Fe 3+ from both experimental [6] , [8] and theoretical [7] studies (red dotted line, Fig. 2a ) is more than twice our observed values. The weighted mean QS for Fe 2+ in all samples increases dramatically with pressure ( Fig. 2b ), which arises from a decreasing intensity of the low QS Fe 2+ doublet (blue doublet in Fig. 1 ) corresponding to the HS state [14] , and an increasing intensity of the high QS doublet (black doublet in Fig. 1 ), which we assign to the IS state [14] , [15] . 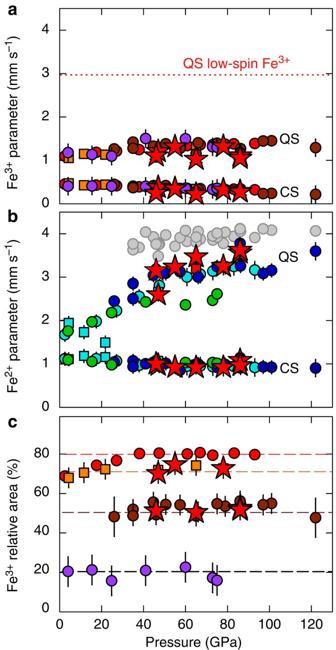Figure 2: Pressure variation of FeAlPv hyperfine parameters. Values of centre shift (CS) and quadrupole splitting (QS) are shown for (a) HS Fe3+and (b) Fe2+. Sample data are indicated as follows: Mg0.6Fe0.4Si0.63Al0.37O3perovskite sample no. 1 (red and light blue circles); Mg0.6Fe0.4Si0.63Al0.37O3perovskite sample no. 2 (orange and light blue squares); Mg0.83Fe0.2Al0.06Si0.91O3perovskite sample no. 3 (brown and dark blue circles); and Mg0.94Fe0.06SiO3perovskite sample no. 4 (purple and green circles). The expected QS for LS Fe3+is shown as a horizontal red dotted line. Hyperfine parameters for Fe2+are shown as weighted averages of the two doublets (colours as above) and QS for the high QS Fe2+doublet (grey circles). (c) Pressure variation of Fe3+/ΣFe as determined from the relative areas in silicate perovskite Mössbauer spectra: sample no. 1 (red circles); sample no. 2 (orange squares); sample no. 3 (brown circles); and sample no. 4 (purple circles). Horizontal lines are guides for the eye. Values obtained after laser heating of samples 2 and 3 are indicated by red stars. Error bars represent 2σ uncertainty based on fitting statistics. In all cases, parameters remained unchanged from those before heating within experimental error, demonstrating that there is no HS to LS transition in Fe3+at the pressure–temperature conditions of the lower mantle. Figure 2: Pressure variation of FeAlPv hyperfine parameters. Values of centre shift (CS) and quadrupole splitting (QS) are shown for ( a ) HS Fe 3+ and ( b ) Fe 2+ . Sample data are indicated as follows: Mg 0.6 Fe 0.4 Si 0.63 Al 0.37 O 3 perovskite sample no. 1 (red and light blue circles); Mg 0.6 Fe 0.4 Si 0.63 Al 0.37 O 3 perovskite sample no. 2 (orange and light blue squares); Mg 0.83 Fe 0.2 Al 0.06 Si 0.91 O 3 perovskite sample no. 3 (brown and dark blue circles); and Mg 0.94 Fe 0.06 SiO 3 perovskite sample no. 4 (purple and green circles). The expected QS for LS Fe 3+ is shown as a horizontal red dotted line. Hyperfine parameters for Fe 2+ are shown as weighted averages of the two doublets (colours as above) and QS for the high QS Fe 2+ doublet (grey circles). ( c ) Pressure variation of Fe 3+ /ΣFe as determined from the relative areas in silicate perovskite Mössbauer spectra: sample no. 1 (red circles); sample no. 2 (orange squares); sample no. 3 (brown circles); and sample no. 4 (purple circles). Horizontal lines are guides for the eye. Values obtained after laser heating of samples 2 and 3 are indicated by red stars. Error bars represent 2σ uncertainty based on fitting statistics. In all cases, parameters remained unchanged from those before heating within experimental error, demonstrating that there is no HS to LS transition in Fe 3+ at the pressure–temperature conditions of the lower mantle. Full size image Our data demonstrate that Fe 3+ A does not undergo a HS to LS transition up to at least 122 GPa. This conclusion is in agreement with results from experimental [6] , [8] and theoretical [4] , [5] , [7] studies. However, several publications [6] , [8] , [9] have suggested that the reduced volume of LS Fe 3+ B could lead to a redistribution of Fe 3+ from the A to the B site in the perovskite structure within the lower mantle. To test this hypothesis, we laser annealed sample no. 2 and 3 at lower-mantle temperatures and a number of pressures and collected SMS spectra both during and after heating. The total duration of heating reached several hours after multiple cycles. Visually, SMS spectra collected after laser annealing showed no change to those taken before heating ( Supplementary Fig. S2 ), and hyperfine parameters remain unchanged (star symbols; Fig. 2 ). We therefore conclude that there is no exchange of Fe 3+ between the A and the B site at lower-mantle pressures and temperatures, in agreement with the results of a complementary study using high-pressure single-crystal X-ray diffraction with laser heating undertaken on the same composition as two of our samples [14] . Electrical conductivity Electromagnetic induction data offer an important complement to seismic data with respect to lower-mantle modelling, because the former are more sensitive to temperature and iron content, whereas the latter better constrain the mineralogy [21] . Laboratory electrical conductivity data of the relevant minerals are an important component of the approach, because they provide critical data on how the chemical and thermal state of the material influences the conductivity. Laboratory measurements of single-phase Mg 0.9 Fe 0.1 SiO 3 perovskite [10] , [11] and a pyrolite mantle assemblage [12] (Fe 3+ /ΣFe of the perovskite phase estimated to be 12% and 30%, respectively) [22] show a decrease in conductivity >50 GPa, comparable to the electrical conductivity decrease caused by HS–LS spin cross-over of Fe 2+ in (Mg,Fe)O(refs 23 , 24 , 25 ). The drop in silicate perovskite conductivity has been attributed to a HS–LS transition of Fe 3+ (refs 10 , 11 , 12 ); however, this explanation is ruled out by the results in the present work. To investigate the relative contributions of Fe 2+ and Fe 3+ , we measured the electrical resistance of Mg 0.6 Fe 0.4 Si 0.63 Al 0.37 O 3 perovskite (93% Fe 3+ /ΣFe) [19] at high pressure and high temperature, which shows a smooth decrease with increasing pressure ( Fig. 3a ). This decrease corresponds to a smooth increase in electrical conductivity with pressure, in contrast to the large drop seen in samples dominated by Fe 2+ ( Fig. 3b ). Such behaviour strongly suggests that the conductivity drop in samples dominated by Fe 2+ is due to the HS to IS transition in Fe 2+ , where electron mobility is reduced due to the spin transition, analogous to the behaviour of (Mg,Fe)O [23] , [24] , [25] . The greater drop at high temperature (brown circles in Fig. 3b ) is consistent with the increasing stability of the IS state with temperature [14] , [15] . 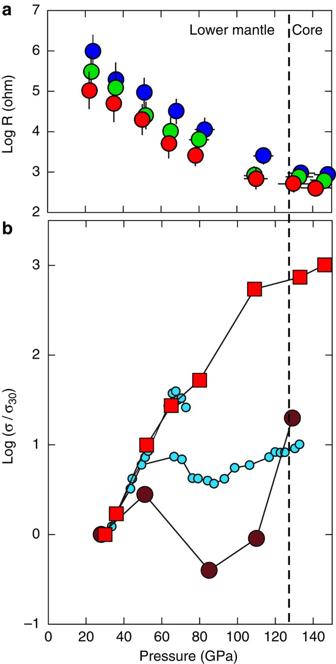Figure 3: Electrical properties of FeAlPv as a function of pressure. (a) Influence of pressure on the electrical resistance of Mg0.60Fe0.40Si0.63Al0.37O3perovskite (Fe3+/ΣFe = 0.93±0.3) measured using a laser-heated DAC at different temperatures: blue —1250±50 K; green —1800±50 K; red —2300±100 K. Error bars represent 2σ uncertainty of the measurement value. (b) Relative change of electrical conductivity of FeAlPv as a function of pressure calculated from resistance data. Red squares indicate new data for Mg0.6Fe0.4Si0.63Al0.37O3perovskite (Fe3+/ΣFe~93%) collected at 1800 K. Also shown are two sets of literature data for Mg0.9Fe0.1SiO3perovskite (Fe3+/ΣFe~12%) at room temperature (blue circles)11and a pyrolite assemblage (Fepv3+/ΣFepv~30%)22at 1800 K (brown circles)12. Data are plotted relative to the values at 30 GPa (σ30). The error bars representing the precision of the data from this work are smaller than the symbols (red squares). Figure 3: Electrical properties of FeAlPv as a function of pressure. ( a ) Influence of pressure on the electrical resistance of Mg 0.60 Fe 0.40 Si 0.63 Al 0.37 O 3 perovskite (Fe 3+ /ΣFe = 0.93±0.3) measured using a laser-heated DAC at different temperatures: blue —1250±50 K; green —1800±50 K; red —2300±100 K. Error bars represent 2σ uncertainty of the measurement value. ( b ) Relative change of electrical conductivity of FeAlPv as a function of pressure calculated from resistance data. Red squares indicate new data for Mg 0.6 Fe 0.4 Si 0.63 Al 0.37 O 3 perovskite (Fe 3+ /ΣFe~93%) collected at 1800 K. Also shown are two sets of literature data for Mg 0.9 Fe 0.1 SiO 3 perovskite (Fe 3+ /ΣFe~12%) at room temperature (blue circles) [11] and a pyrolite assemblage (Fe pv 3+ /ΣFe pv ~30%) [22] at 1800 K (brown circles) [12] . Data are plotted relative to the values at 30 GPa (σ 30 ). The error bars representing the precision of the data from this work are smaller than the symbols (red squares). Full size image Previously temperature and total iron content have been considered to have the greatest influence on lower-mantle electrical conductivity profiles [21] , but our data show that Fe 3+ /ΣFe could also affect conductivity significantly at mid-mantle depths (1200–1900, km). A companion work has shown that Fe 3+ /ΣFe could also affect bulk sound velocity in the lower mantle [19] ; hence, joint inversion of electromagnetic and seismic data based on these new data could yield results different to currently accepted views. For example the superadiabatic temperature gradient inferred for the lower mantle from such a joint inversion [21] may not be required due to the reduced electrical conductivity of silicate perovskite resulting from the HS-IS transition. Three-dimensional inversions of electromagnetic data are now possible, and show variations of more than one order of magnitude in electrical conductivity, many of which are correlated with fast and slow regions of seismic tomography models [26] . Our new data suggest that for silicate perovskite with lower-mantle composition, a lower Fe 3+ /ΣFe ratio will cause lower conductivity (reduction of conductivity due to the Fe 2+ HS-IS transition) and a higher bulk sound velocity [19] . Indeed many regions were found to show such a correlation [26] , which could be indicative of bulk mantle properties away from areas associated with subduction. In conclusion, based on novel SMS data we have demonstrated the absence of a spin transition of Fe 3+ in FeAlPv at pressures and temperatures corresponding to those in the lower mantle. Electrical conductivity measurements of Fe 3+ -rich FeAlPv show no evidence for the conductivity drop previously observed in Fe 2+ -rich FeAlPv compositions, suggesting that the conductivity drop is due to the reduced mobility of electrons caused by a HS-IS transition of Fe 2+ . Combined with recent results reporting the influence of Fe 3+ on elastic wave velocities of FeAlPv, our results may provide improved constraints for forward modelling of electromagnetic data as well as for joint inversion of electromagnetic and seismic data, potentially providing a new probe of heterogeneity in the lower mantle. Synchrotron Mössbauer source A SMS provides a high-brilliance beam of synchrotron radiation with an energy bandwidth of ~20 neV. The SMS beam is polarized up to 99%, and it consists 100% of recoilless radiation with zero background. These properties enable rapid and precise measurements of Mössbauer spectra of samples under extreme conditions. The possibility to develop such a source was first demonstrated at the Nuclear Resonance beamline ID18 (ref. 27 ) at the European Synchrotron Radiation Facility in 1997 (ref. 28 ), and technical details of the configuration used in the present work are given in Potapkin et al. [18] ) 57 Fe SMS spectra were collected on the nuclear resonance beamline ID18 at the European Synchrotron Radiation Facility during operation in multibunch mode (7/8+1 filling) with the beam focused to roughly 10 × 10 μm 2 using Kirkpatrick–Baez multilayer optics. During the SMS experiment, the linewidth of the source was controlled before and after each sample measurement using K 2 Mg 57 Fe(CN) 6 , whose Mössbauer spectrum consists of a single line, and the velocity scale was calibrated using 25-μm thick natural α-iron foil. SMS spectra were collected over 10–60 min each. Spectra were fitted using the program MossA [29] , which takes into account the Lorentzian-squared source instrumental function [30] . The dimensionless effective Mössbauer thicknesses were approximately 40 and 20 for the Mg 0.6 Fe 0.4 Si 0.63 Al 0.37 O 3 perovskite sample no. 1 and 2, and 8 and 3 for the Mg 0.83 Fe 0.2 Al 0.06 Si 0.91 O 3 and Mg 0.94 Fe 0.06 SiO 3 perovskite samples, respectively. Sample synthesis All silicate perovskite samples were synthesized using a multianvil press. The experiments were performed using Cr 2 O 3 -doped MgO octahedra fitted with a LaCrO 3 heater in combination with tungsten carbide cubes following the methodology described in Keppler and Frost [31] . Chemical compositions were measured using an electron microprobe (S4949 and S5083) or estimated based on electron microprobe measurements of a sample synthesied under the same conditions in a different run (S4850). Details of each experiment are given in Table 1 . DAC experiments Samples for DAC experiments were carefully selected from the run products to be homogeneous under an optical microscope. Small plate-like pieces of the material (typical dimensions ~30 × 30 × 15 μm 3 ) were loaded together with ruby chips (pressure marker) into the sample chambers of DACs available at Bayerisches Geoinstitut. Diamonds with culets of diameter 120, 250 and 300 μm were used in different experiments depending on the pressure range. The sample chamber was prepared by drilling a hole in a pre-indented rhenium gasket, and the hole was filled with the sample material and the quasi-hydrostatic pressure medium, Ne. We used a modified and enhanced version of the portable laser heating setup described previously [32] , [33] . The setup was installed on beamline ID18 and consists of a SPI laser system (SPI100, wavelength 1064, nm, 100 W) coupled by an optical fibre to a UniHead system, which allows simultaneous visual observation of the sample, laser heating and evaluation of temperature. In order to ensure homogeneous heating of the samples, a laser spot with a diameter of about 50 μm was used. In order to guarantee homogeneous heating, we flattened the power profile of the laser beam using a special optical device ( π -shaper) mounted on the UniHead. Samples 2 and 3 were heated for a total of several hours in multiple cycles during continuous laser operation mode. Thermal radiation from the heated sample was collected by an Ocean Optics QE65000 spectrometer, and the resulting spectra were fitted to the Planck radiation function [34] , which gave temperatures between 2000 and 2400 K. SMS spectrum fitting SMS spectra can be fitted using the same approach for conventional energy-domain Mössbauer spectra provided the following criteria are met: (a) the source lineshape is implemented as a normalized squared Lorentzian (instead of a normalized Lorentzian) [30] ; (b) the full transmission integral is used to fit the data because of the high absorption and the lack of non-resonant background; and (c) component areas of doublets and sextets are not fixed to ideal values (that is, 1:1 for quadrupole doublets and 3:2:1:1:2:3 for magnetic sextets) because of the polarized nature of the synchrotron source combined with the tendency for preferred orientation in the DAC. We fit all of the SMS spectra to three quadrupole doublets, one with small centre shift (average value ~0.35 mm s −1 ) corresponding to Fe 3+ , and two with larger centre shift (average value ~1 mm s −1 ) corresponding to Fe 2+ . We applied the conventional constraint of equal widths but allowed the area ratios of component doublets to vary, with all area ratios of doublets within a single spectrum constrained to be the same based on the reasonable assumption that the principal directions of the electric-field gradient for both the A and the B sites are the same based on the crystallography of the perovskite structure. Electrical conductivity measurements Resistance measurements were conducted at high pressure and high temperature on a sample of Mg 0.60 Fe 0.40 Si 0.63 Al 0.37 O 3 perovskite (Fe 3+ /ΣFe=0.93±0.3) that was synthesized in a multianvil run using the same starting materials and at the same conditions as samples 1 and 2. We used a BX90-type DAC [35] where a standard brilliant cut diamond with 400 μm culet was used as the first anvil, and a conventional beveled diamond with 120 μm culet was used as the second anvil. To prepare the gasket, a 50-μm diameter hole was drilled in a 25-μm thick piece of rhenium foil, after which the drilled piece of rhenium was cut into two halves using a near-infrared laser with the cutting plane passing through the middle of the hole. The two rhenium foil halves were coated with a gold layer roughly 2-μm thick using a simple sputter coater and then glued onto a synthetic single-crystal diamond, thus providing a split-gasket hole configuration for the sample chamber. A platinum wire with 20 μm diameter was used in a linear four-point probe scheme (see Kuznetsov et al. [36] for technical details). Current was supplied through two platinum leads glued onto different halves of the split gasket, and voltage was measured using the other two leads. The particular construction of the DAC used enabled the platinum leads from the gasket to emerge freely from the DAC to then be connected to measuring devices, whereas thin ceramic tubes prevented potential contact of the platinum wires with the metallic body of the DAC. Small pieces of sample roughly 10–12 μm in diameter and 5–7-μm thick were loaded into the middle of the split-gasket hole. Synthetic diamond powder (grain size <1 μm) placed in the slits between the halves of the split gasket provided reliable insulation of the two halves of the gasket, whereas the sample in the split-gasket hole closed the circuit. The current and voltage measurements were read out using multimeters. The sample was heated using a portable laser heating system as previously described [32] . Resistance data were collected at pressures up to 146 GPa at three different temperatures (1250, 1800 and 2300 K). The quantity σ/σ 30 (that is, the electrical conductivity relative to the value at 30 GPa) was calculated based on the change in height of the sample as a function of pressure that was measured in a separate experiment. How to cite this article: Potapkin, V. et al. Effect of iron oxidation state on the electrical conductivity of the Earth’s lower mantle. Nat. Commun. 4:1427 doi: 10.1038/ncomms2436 (2013).